TALEN and CRISPR/Cas9-mediated genome editing in the early-branching metazoanNematostella vectensis Non-bilaterian phyla represent key lineages for exploring the evolutionary history of early animals. However, despite an increasing number of sequenced genomes from early-branching metazoans, efficient and reproducible methodologies for analysis of gene function remain a major challenge. Here we report the utilization of the TALEN and CRISPR/Cas9 systems to induce targeted mutations and homologous recombination-mediated transgenesis in the sea anemone Nematostella vectensis . We also present a new method to isolate genetically modified animals using engineered selection cassettes introduced by homologous recombination. Taken together, these methods will permit sophisticated gain- and loss-of-function analyses in Nematostella and perhaps other early metazoan species that allow for zygotic injection. The recent advent of genome-editing tools promises to democratize the molecular-genetic interrogation of animal biology, in both basic and biomedical applications. To date, transcription activator-like effector nucleases [1] , [2] (TALENs) and the clustered regulatory interspaced short palindromic repeats-associated endonuclease Cas9 (refs 3 , 4 ) (CRISPR/Cas9) have been applied to edit the genome in cell culture [5] , [6] , [7] and a few select model organisms from the bilaterian clade [8] , [9] , [10] , [11] . Among the non-bilaterians (Cnidaria, Placozoa, Porifera and Ctenophora), experimental tools remain a limiting factor for functional studies, restricting the available approaches to partial and imprecise gene disruption via morpholinos, RNA interference, pharmacological inhibitor experiments and correlative analyses of gene expression patterns. Thus, for studies of early animal evolution and development, genome-editing methods now present a transformative opportunity to manipulate gene function in vivo . The genome of the cnidarian Nematostella vectensis was the first to be sequenced among the early Metazoa [12] , revealing an unexpected degree of genetic complexity in what was once regarded as a ‘primitive’ animal. Combined with its phylogenetic position, extensive regenerative capacity and relative ease of laboratory spawning, Nematostella has become a highly attractive model for comparative genomics and evolutionary developmental biology [13] . Although morpholino-mediated knockdown [14] , injection of messenger RNA (mRNA) [15] and meganuclease-mediated transgenesis [16] methods have been applied in Nematostella , their utility is generally restricted to early embryonic development or subject to considerable functional limitations. Here, to expand the experimental toolkit in Nematostella while establishing a proof of principle for all early metazoan systems, we report methods to perform precise in vivo gene editing using both TALEN- and CRISPR/Cas9-mediated homologous recombination. We first employ the TALEN and CRISPR/Cas9 systems to generate targeted mutations in NvFP-7R , a locus encoding an endogenous Nematostella red fluorescent protein [17] . Second, we develop an efficient method to track genomic lesions in both somatic and germline cells with selection cassettes introduced through TALEN and CRISPR/Cas9-mediated homologous recombination. Finally, using NvFP-7R as a landing site, we establish a robust homologous recombination-mediated transgenesis method for Nematostella . TALEN-mediated mutagenesis at the NvFP-7R locus To generate site-directed mutations likely to yield clear but non-lethal phenotypes, we targeted an endogenous Nematostella red fluorescent protein (NvFP-7R) using the TALEN system. We previously reported that NvFP-7R encodes a red fluorescent protein that is specifically expressed in the oral pole of adult polyps [17] ( Fig. 1a ). We thus constructed a TALEN pair that recognizes a target sequence within the obligate second exon of NvFP-7R (NvFP-7R-TALEN; Fig. 1b ). Taking advantage of the fact that the Nematostella genome contains seven green fluorescent protein (GFP)-like genes, we also used BLAST to characterize putative off-target sites in NvFP5 and NvFP4 . These loci exhibited either two or six nucleotide mismatches in the TALEN target site, respectively ( Supplementary Fig. 1a ), and thus provided an internal control for TALEN specificity. 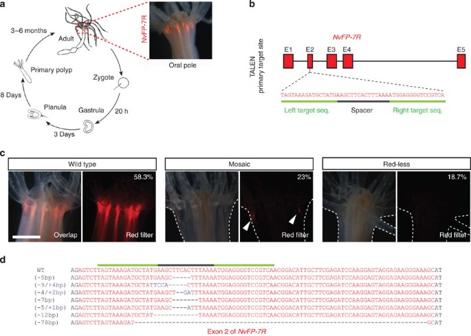Figure 1: TALEN-induced mutations inNvFP-7R. (a) The life cycle ofNematostella. After fertilization, embryos undergo gastrulation and develop into swimming planulae that give rise to four-tentacle primary polyps. Primary polyps begin feeding and grow to form 16-tentacle adults. At the 12-tentacle stage (~1.5 months),Nematostellaspecifically express NvFP-7R at the oral pole (inset box). (b) Gene model ofNvFP-7Rshowing the target site of the NvFP-7R-TALEN pair in exon 2 (E2). TALEN-binding sites are underlined in green. The spacer sequence is underlined in black. (c) TALEN-injected animals exhibit three phenotypes ofNvFP-7Rexpression. The first phenotype appears normal (wild type). The second phenotype (mosaic) displays loss of NvFP-7R expression in one or more domains and normal expression in others (white arrowheads). The third phenotype lacks any detectable expression ofNvFP-7R(red-less). The percentages of each phenotype are indicated (n=312). Dotted lines indicate the outline of the oral pole. Scale bar, 1 mm. (d) Molecular characterization of NvFP-7R-TALEN-induced mutations recovered from a phenotypically Red-less F0 animal. Figure 1: TALEN-induced mutations in NvFP-7R . ( a ) The life cycle of Nematostella . After fertilization, embryos undergo gastrulation and develop into swimming planulae that give rise to four-tentacle primary polyps. Primary polyps begin feeding and grow to form 16-tentacle adults. At the 12-tentacle stage (~1.5 months), Nematostella specifically express NvFP-7R at the oral pole (inset box). ( b ) Gene model of NvFP-7R showing the target site of the NvFP-7R-TALEN pair in exon 2 ( E2 ). TALEN-binding sites are underlined in green. The spacer sequence is underlined in black. ( c ) TALEN-injected animals exhibit three phenotypes of NvFP-7R expression. The first phenotype appears normal (wild type). The second phenotype (mosaic) displays loss of NvFP-7R expression in one or more domains and normal expression in others (white arrowheads). The third phenotype lacks any detectable expression of NvFP-7R (red-less). The percentages of each phenotype are indicated ( n =312). Dotted lines indicate the outline of the oral pole. Scale bar, 1 mm. ( d ) Molecular characterization of NvFP-7R-TALEN-induced mutations recovered from a phenotypically Red-less F0 animal. Full size image Following in vitro transcription from plasmid templates, we microinjected equal amounts of both left and right TALEN mRNAs into unfertilized Nematostella eggs (200 ng μl −1 each; n =803). After fertilization, ~54% of TALEN-injected embryos survived to the primary polyp stage and appeared morphologically normal ( Supplementary Table 1 ). To assay disruption of NvFP-7R , we reared injected animals beyond the 12-tentacle stage when the expression of the endogenous red fluorescence becomes clearly visible [17] . Using a fluorescent dissecting microscope, we identified a high percentage of adult polyps that showed either mosaic (23%) or complete loss (18.7%) of the normal red fluorescence ( Fig. 1c ; Supplementary Fig. 2 ; Supplementary Table 1 ). In these cases, the disruption of red fluorescence was most likely due to biallelic TALEN-induced mutagenesis in a large population of cells. To confirm this, we cloned and sequenced 500 base pairs of genomic DNA, including exon 2, from two ‘red-less’ animals with no detectable NvFP-7R expression. As expected, almost all sequenced NvFP-7R alleles (80 and 100%) carried insertion/deletion mutations at the TALEN target site ( Fig. 1d ). The spectrum of mutation events recovered within individual red-less animals suggests that they originated from independent TALEN-induced double-strand break events followed by errors in non-homologous end joining-mediated repair. Collectively, these findings demonstrate that TALENs can efficiently generate targeted lesions in the Nematostella genome, frequently disrupting both alleles in a large number of somatic cells. NvFP-7R is dispensable for Nematostella development To investigate the function of NvFP-7R in Nematostella , we performed phenotypic analyses of NvFP-7R mutants. At the cellular level, the expression of NvFP-7R is restricted to the endodermal cells between tentacles and the myoepithelial cells of the mesenteries [17] ( Supplementary Fig. 3a–d ), with a significant accumulation of the protein in the contractile elements ( Supplementary Fig. 3e ). In optical cross-sections through the oral region, we observed that polyps exhibiting NvFP-7R loss-of-function were morphologically indistinguishable from wild-type controls ( Supplementary Fig. 3c,d ). More specifically, we did not detect any developmental defects in muscle filaments ( Supplementary Fig. 3e ) or changes in their contractile behaviour ( Supplementary Fig. 3f ; Supplementary Movies 1 and 2 ). Together, these results suggest that NvFP-7R is not required for normal development or homeostasis of Nematostella under laboratory conditions. Germline transmission of TALEN-induced mutations Using a standardized protocol, Nematostella females can be induced to spawn hundreds of eggs clustered in a gelatinous mass. To determine whether TALEN-induced mutations were transmitted through the germline of injected F0 females, we reared them to sexual maturity and then genotyped unfertilized oocytes. By sequencing exon 2 of NvFP-7R , we determined the nature and frequency of TALEN-induced mutations present in the gametes. We did not detect germline mutations in TALEN-injected animals displaying wild-type expression of NvFP-7R ( n =5). In contrast, we documented germline transmission of induced mutations in unfertilized eggs from 50% of red-less F0 females ( n =12; Supplementary Fig. 4a,b ), with a frequency of NvFP-7R mutation up to 80% ( Supplementary Fig. 4c ). These results demonstrate efficient TALEN-induced mutations of the Nematostella germline. Importantly, they also illustrate how the presence of a visible marker can significantly increase the probability of identifying founder animals. As a general strategy for TALEN-mediated mutagenesis, the use of visual selection cassettes could greatly facilitate the isolation of genetically modified individuals. TALEN-mediated homologous recombination at the NvFP-7R locus In a limited number of cases, TALEN-mediated homologous recombination has been used to insert exogenous DNA into the genomes of Drosophila [11] , zebrafish [8] and mouse [18] . To test this approach as a means to insert a selection cassette in Nematostella NvFP-7R , we constructed a donor vector containing two distinct selection markers flanked by one kilobase (kb) of left and right genomic homology arms ( Fig. 2a ). The first selection marker comprised the coding sequence for mCherry under the control of the myosin heavy chain1 ( MHC1) promoter, which drives expression in muscle cells [16] ( MHC1-mCherry ). The second selection marker was a protein trap reporter designed to insert enhanced GFP (eGFP) in frame with NvFP-7R exon 2 upon successful integration ( NvFP-7R::eGFP ). Hypothetically, when this dual reporter cassette integrates into the TALEN-exon2 target site, we expect to see both: (1) stable expression of MHC1-mCherry ; and (2) replacement of the red fluorescence of NvFP-7R by the expression of a green NvFP-7R::eGFP fusion protein at the oral end of adult animals ( Fig. 2b ). 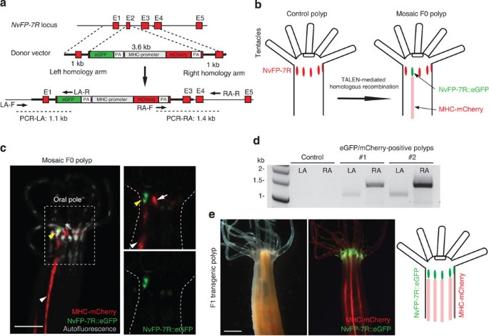Figure 2: TALEN-mediated homologous recombination at theNvFP-7Rlocus. (a) Schematic representation ofNvFP-7R, theNvFP-7R::eGFP–MHC-mCherryselection cassette with homology arms (bold lines), and the expected product of TALEN-mediated homologous recombination. (b) Schematic representation of the oral pole of a control polyp and a F0 polyp showing the expected mosaic substitution ofNvFP-7Rby theeGFPfusion cassette withMHC-mCherry. (c) Confocal image of a representative eGFP/mCherry-positive animal co-injected with TALENs and theNvFP-7R::eGFP–MHC-mCherrydonor plasmid. Notice that the large clone of mCherry-positive cells (white arrowhead) also exhibits a replacement ofNvFP-7RbyeGFP(yellow arrowhead). Only one domain displaying normal expression ofNvFP-7Ris maintained in this polyp (white arrow). Asterisk indicates the position of the mouth. Dotted lines indicate the outline of the oral pole. Scale bar, 500 μm. (d) PCR analysis of TALEN-mediated homologous recombination at theNvFP-7Rlocus in two eGFP/mcherry-positive polyps (#1 and #2). Primers pairs and expected PCR products for the left (LA) and right (RA) arms are indicated ina. (e) A F1 transgenic polyp exhibiting a replacement ofNvFP-7Rby theeGFPfusion cassette in allNvFP-7R-expressing cells. Scale bar, 1 mm. Figure 2: TALEN-mediated homologous recombination at the NvFP-7R locus. ( a ) Schematic representation of NvFP-7R , the NvFP-7R::eGFP–MHC-mCherry selection cassette with homology arms (bold lines), and the expected product of TALEN-mediated homologous recombination. ( b ) Schematic representation of the oral pole of a control polyp and a F0 polyp showing the expected mosaic substitution of NvFP-7R by the eGFP fusion cassette with MHC-mCherry . ( c ) Confocal image of a representative eGFP/mCherry-positive animal co-injected with TALENs and the NvFP-7R::eGFP–MHC-mCherry donor plasmid. Notice that the large clone of mCherry-positive cells (white arrowhead) also exhibits a replacement of NvFP-7R by eGFP (yellow arrowhead). Only one domain displaying normal expression of NvFP-7R is maintained in this polyp (white arrow). Asterisk indicates the position of the mouth. Dotted lines indicate the outline of the oral pole. Scale bar, 500 μm. ( d ) PCR analysis of TALEN-mediated homologous recombination at the NvFP-7R locus in two eGFP/mcherry-positive polyps (#1 and #2). Primers pairs and expected PCR products for the left (LA) and right (RA) arms are indicated in a . ( e ) A F1 transgenic polyp exhibiting a replacement of NvFP-7R by the eGFP fusion cassette in all NvFP-7R -expressing cells. Scale bar, 1 mm. Full size image To determine the optimal concentration of donor DNA for TALEN-mediated homologous recombination, we co-injected the NvFP-7R-TALEN mRNAs with varying amounts of circular donor vector into one-cell-stage embryos (10, 80 and 250 ng μl −1 ). Controls injected with the donor vector alone did not show eGFP expression at the 12-tentacle stage, although we did find two rare mCherry-positive polyps (0.5%; n =401) ( Supplementary Table 2 ). In contrast, 4.6% of surviving animals co-injected with TALENs and 80 ng μl −1 of the donor plasmid exhibited large clones of stable mCherry expression in muscle cells ( Supplementary Table 2 ; n =410 polyps). Further, 5/19 of these mCherry-positive animals displayed a substitution of the endogenous red fluorescence by green fluorescence at the 12-tentacle stage ( Fig. 2c ; Supplementary Table 2 ). Because these reporters are only expressed in a subset of cells, this result indicates successful insertion of the selection cassette in at least 1% of surviving polyps. Interestingly, we observed ectopic expression of eGFP in discrete regions around the mouth in almost all mCherry/eGFP-positive polyps ( Supplementary Fig. 5 ), possibly due to disruption of the NvFP-7R regulatory architecture by the 3.6-kb cassette. To molecularly characterize integration events, we PCR-screened two eGFP–MHC1-mCherry-positive animals using primers within the selection cassette paired with genomic primers positioned outside the homology arms ( Fig. 2a ). As expected, we obtained PCR products of the correct size and sequence ( Fig. 2d ), confirming TALEN-mediated homologous recombination in Nematostella somatic cells. By individually outcrossing three F0 founders with large mCherry/eGFP-positive clones, we observed germline transmission of the selection cassette in the progeny of two ( Fig. 2e ). Insertion of a heat shock-inducible reporter in NvFP-7R To build a selection cassette hypothetically inducible in all cells, we generated a donor vector containing a heat-shock-inducible reporter ( hs-eGFP ) flanked by NvFP-7R left and right homology arms each comprising 2 kb of cloned genomic sequence. Within the selection cassette, eGFP is driven by the Nematostella heat-shock protein 70 promoter (HSP70p), which was identified through homology with the vertebrate HSP70p ( Fig. 3a ). Confirming its function, this promoter induced robust expression of eGFP in injected embryos that were incubated for 30 min at 37 °C ( Fig. 3b ). After injection of the NvFP-7R-TALEN mRNAs and the hs-eGFP selection cassette into Nematostella embryos, 434 injected animals were grown to sexual maturity and spawned to examine their offspring. After a 30-min heat shock at 37 °C, we observed numerous eGFP-positive embryos in the F1 progeny, demonstrating germline transmission of the selection cassette ( Fig. 3c ). Amplification and sequencing of the DNA regions flanking the insertion confirmed that genomic integration occurred at the expected TALEN-exon2 target site ( Fig. 3d ). By analysing F0 adult polyps lacking red fluorescence at the oral pole, we further enriched for disruption of NvFP-7R . In independent spawning of the same animals, 1/20 and 1/8 red-less adults exhibited germline transmission of the hs-eGFP selection cassette. Taken together, these results show that TALEN-mediated homologous recombination functions in both somatic and germline cells and can be used to introduce exogenous sequences into target sites in the Nematostella genome. 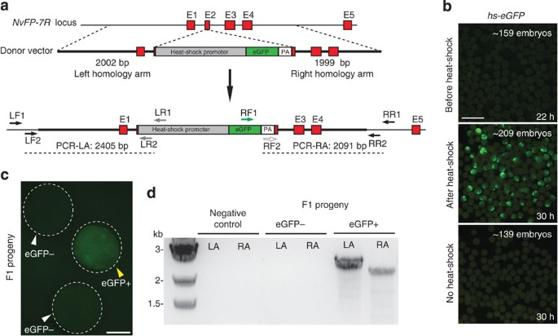Figure 3: TALEN-mediated homologous recombination at theNvFP-7Rlocus using thehs-eGFPdonor vector. (a) Schematic representation of thehs-eGFPselection cassette with homology arms. The expected result of TALEN-mediated homologous recombination is also shown in the scheme. (b)hs-eGFP-injected embryos show strong expression of eGFP after heat-shock treatment (30 min at 37 °C), but not those incubated at room temperature. Scale bar, 600 μm. (c) Three F1 embryos spawned by red-less females co-injected withNvFP-7R-TALENsand thehs-eGFPdonor vector. Yellow arrowhead indicates a representative F1 eGFP-positive embryo. Notice that the expression level of eGFP in the F0 injected-embryos is stronger than that observed in the F1 progeny. This is most likely due to the presence of a single copy ofhs-eGFPin F1 embryos. Scale bar, 100 μm. (d) PCR analysis of TALEN-mediated homologous recombination at theNvFP-7Rlocus in eGFP+and eGFP−embryos (n=5 each). Primers pairs and expected PCR products are indicated ina. Figure 3: TALEN-mediated homologous recombination at the NvFP-7R locus using the hs-eGFP donor vector. ( a ) Schematic representation of the hs-eGFP selection cassette with homology arms. The expected result of TALEN-mediated homologous recombination is also shown in the scheme. ( b ) hs-eGFP -injected embryos show strong expression of eGFP after heat-shock treatment (30 min at 37 °C), but not those incubated at room temperature. Scale bar, 600 μm. ( c ) Three F1 embryos spawned by red-less females co-injected with NvFP-7R-TALENs and the hs-eGFP donor vector. Yellow arrowhead indicates a representative F1 eGFP-positive embryo. Notice that the expression level of eGFP in the F0 injected-embryos is stronger than that observed in the F1 progeny. This is most likely due to the presence of a single copy of hs-eGFP in F1 embryos. Scale bar, 100 μm. ( d ) PCR analysis of TALEN-mediated homologous recombination at the NvFP-7R locus in eGFP + and eGFP − embryos ( n =5 each). Primers pairs and expected PCR products are indicated in a . Full size image Off-target activity of TALENs in Nematostella The NvFP-7R-TALEN pair utilized in this study could potentially recognize secondary sites in two related fluorescent proteins. We took advantage of this to characterize off-target effects in red-less animals exhibiting a high degree of NvFP-7R disruption. Intriguingly, the NvFP5 site containing two mismatches was mutated in all analysed animals ( n =3), but we did not detect any mutations in the NvFP4 site, which includes six mismatches ( Supplementary Fig. 1b ). Consistent with a previous report [19] , this suggests that TALENs can tolerate two mismatches in vivo . This could be advantageous for simultaneous disruption of multiple members of a gene family to examine phenotypes obscured by functional redundancy. Further, it also suggests a minimal guideline for avoiding undesired off-target cleavage events in Nematostella . CRISPR/Cas9-mediated gene editing in Nematostella The construction of functional TALEN pairs can be challenging and time-consuming. As an alternative, the CRISPR/Cas9 system is a more flexible and cost-effective method for genome editing based on RNA-guided endonuclease activity [20] . To establish this method in Nematostella , we designed two guide RNAs (gRNAs) that target 20-bp sequences in exons 2 and 3 of NvFP-7R (gRNA- NvFP-7R Exon2 and gRNA- NvFP-7R Exon3 ; Fig. 4a ). To validate the functionality of our gRNA–Cas9 complexes in vitro , we analysed their capacity to direct recombinant Cas9 to cut the correct target sequence ( Fig. 4a ). Both gRNA–Cas9 complexes produced the expected DNA fragments from a linearized plasmid, indicating that they successfully cleaved their corresponding target sites ( Fig. 4b ). To test this approach in vivo , we injected an in vitro assembled gRNA-Exon2/Cas9 complex into unfertilized eggs. Strikingly, 10% of the resulting adult polyps exhibited mosaic red fluorescent protein expression ( n =532; Supplementary Table 3 ). We confirmed mutagenesis of the expected site in NvFP-7R in each of three mosaic 12-tentacle polyps analysed ( Fig. 4c ). 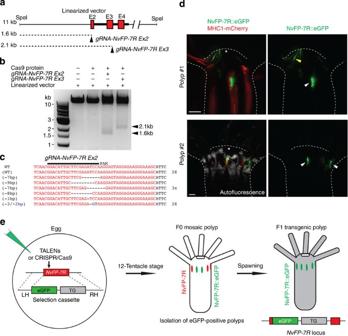Figure 4: CRISPR/Cas9-mediated editing ofNvFP-7R. (a) Schematic representation of a linearized plasmid containing 2 kb of theNvFP-7Rlocus, including thegRNA-NvFP-7R Exon2andgRNA-NvFP-7R Exon3target sites (black arrowheads). The short DNA fragments (dotted lines) expected after Cas9-mediated cleavage by each gRNA are 1.6 and 2.1 kb, respectively. (b)In vitroDNA cleavage assay using recombinant Cas9 with gRNAs. Negative controls are the linearized plasmid alone or with Cas9 protein. Both gRNA/Cas9 complexes generated the expected DNA fragments (black arrowheads). (c) gRNA-NvFP-7R Exon2/Cas9-induced mutations recovered from a single polyp that exhibited mosaic expression ofNvFP-7R. The back line indicates the target site of gRNA-NvFP-7R Exon2with its PAM sequence. (d) Confocal image of two representative eGFP/mcherry-positive animals co-injected with anin vitroassembled gRNA-Exon2/Cas9 complex and a variant of theNvFP-7R::eGFP–MHC-mCherrydonor plasmid. Polyp #1 displays a substitution ofNvFP-7RbyNvFP-7R::eGFPin one domain, while polyp #2 shows two domains ofNvFP-7R::eGFPexpression (white arrowheads). Polyp #1 also exhibits ectopic expression ofNvFP-7R::eGFP(yellow arrowhead). Asterisk (*) indicates the position of the mouth. Scale bar, 100 μm. (e) Workflow for homologous recombination-mediated transgenesis inNematostellabased on the conversion of the endogenous red fluorescence into eGFP. The ease of visual screening allows efficient isolation of precise genomic integration of a transgene (TG,grey). Figure 4: CRISPR/Cas9-mediated editing of NvFP-7R . ( a ) Schematic representation of a linearized plasmid containing 2 kb of the NvFP-7R locus, including the gRNA-NvFP-7R Exon2 and gRNA-NvFP-7R Exon3 target sites (black arrowheads). The short DNA fragments (dotted lines) expected after Cas9-mediated cleavage by each gRNA are 1.6 and 2.1 kb, respectively. ( b ) In vitro DNA cleavage assay using recombinant Cas9 with gRNAs. Negative controls are the linearized plasmid alone or with Cas9 protein. Both gRNA/Cas9 complexes generated the expected DNA fragments (black arrowheads). ( c ) gRNA- NvFP-7R Exon2 /Cas9-induced mutations recovered from a single polyp that exhibited mosaic expression of NvFP-7R . The back line indicates the target site of gRNA- NvFP-7R Exon2 with its PAM sequence. ( d ) Confocal image of two representative eGFP/mcherry-positive animals co-injected with an in vitro assembled gRNA-Exon2/Cas9 complex and a variant of the NvFP-7R::eGFP–MHC-mCherry donor plasmid. Polyp #1 displays a substitution of NvFP-7R by NvFP-7R::eGFP in one domain, while polyp #2 shows two domains of NvFP-7R::eGFP expression (white arrowheads). Polyp #1 also exhibits ectopic expression of NvFP-7R::eGFP (yellow arrowhead). Asterisk (*) indicates the position of the mouth. Scale bar, 100 μm. ( e ) Workflow for homologous recombination-mediated transgenesis in Nematostella based on the conversion of the endogenous red fluorescence into eGFP. The ease of visual screening allows efficient isolation of precise genomic integration of a transgene (TG, grey ). Full size image To assay for CRISPR/Cas9-mediated homologous recombination, we also co-injected the gRNA-Exon2 /Cas9 complex with a variant of the NvFP-7R::eGFP–MHC1-mCherry selection cassette described above. Here, 6.4% of surviving 12-tentacle polyps displayed the expression of mCherry, and 18.7% of these animals were also NvFP-7R::eGFP-positive, consistent with integration at the correct genomic site ( Supplementary Table 2 ). Intriguingly, NvFP-7R::eGFP expression was once again detected at ectopic positions around the oral pole ( Fig. 4d ), similar to the effect we observed following TALEN-mediated homologous recombination at a different position in exon 2 ( Supplementary Fig. 5 ). This reinforces the hypothesis that cassette integration disrupts transcriptional regulation of the NvFP-7R locus. In parallel with the experiments above, we tested the efficiency of the CRISPR/Cas9 system using injection of Cas9 mRNA instead of recombinant Cas9 protein. To do so, we employed the self-cleaving 2A peptide [21] , [22] to generate a bicistronic construct encoding nuclear eGFP and Cas9 under the control of the SP6 promoter ( nls-eGPF-2A-Cas9 ; Supplementary Fig. 6a,b ). After injection of the nls-eGPF-2A-Cas9 mRNA (250 ng μl −1 ) into unfertilized eggs, we detected nuclear eGFP at 4 h post fertilization (h.p.f.) and its expression level increased 30-fold reaching a plateau around 19 h.p.f. ( Supplementary Fig. 6b,c ; Supplementary Movie 3 ). Following co-injection of nls-eGPF-2A-Cas9 mRNA, gRNA-Exon2 and the NvFP-7R::eGFP–MHC1-mCherry plasmid into Nematostella eggs, 16.8% of primary polyps exhibited mosaic expression of mCherry ( n =434). We molecularly confirmed the integration of the cassette at the expected target site in two primary polyps ( Supplementary Fig. 6d ). Although the frequency of mCherry-positive polyps was higher after the injection of Cas9 mRNA, it is noteworthy that the sizes of the mCherry-positive clones were generally smaller than those recovered in recombinant Cas9 protein-injected animals. We speculate that the presence of Cas9 protein during initial cleavage stages may allow early integration events. To extend the CRISPR/Cas9-mediated homologous recombination approach to another locus, we designed a gRNA targeting a sequence in the first exon of Nvanthox6 ( gRNA-hox6 ). We also generated a donor vector containing the MHC1-mCherry selection cassette flanked by 1.4 kb of Nvanthox6 left and right genomic homology arms ( Supplementary Fig. 7a ). Following co-injection of this donor vector with gRNA-hox6 /Cas9 protein complex, 4.5% of recovered polyps were mCherry-positive ( n =440), and we molecularly validated the disruption of Nvanthox6 exon 1 by the MHC1-mCherry cassette in a pool of five F0 primary polyps ( Supplementary Fig. 7b ). On the basis of the analysis of two independent loci, our results demonstrate a specific methodology by which the CRISPR/Cas9 system can be used to induce and select for site-specific DNA modifications in Nematostella . While additional analysis would be required to characterize potential off-target effects of the CRISPR/Cas9 system, these methods open the door to a wide range of functional manipulations in vivo . In summary, we have demonstrated the utility of integrated selection cassettes for the identification of TALEN- and CRISPR/Cas9-induced mutations in an early metazoan. This approach, which should be widely applicable, allows for the rapid isolation of both somatic and germline mutations based on visible markers. Using this general strategy, it should be possible to mutate, tag or otherwise modify any target sequence in the Nematostella genome. Following from this proof of principle, the same experimental approach has the potential to succeed in any non-bilaterian system with accessible eggs. In Nematostella , we propose the use of NvFP-7R as a landing site for TALEN or CRISPR/Cas9-mediated transgenesis. As a visible readout of transgene insertion, cassette-mediated conversion of NvFP-7R into NvFP-7R::eGFP allows for efficient isolation of precise genomic integration events ( Fig. 4e ). Besides the ease of visual screening, this approach eliminates concern over position effects and multicopy insertions that could occur in the traditional meganuclease-mediated transgenesis method. On a general note, a broad effort is underway to reconstruct the evolution of animal complexity through comparative studies of phylogenetically informative lineages, including cnidarians [23] , [24] , [25] , ctenophores [26] , [27] , placozoans [28] , [29] and sponges [30] , [31] . While sequencing projects have produced an abundance of information about the genomic foundations of animal evolution [32] , emerging genetic tools of the kind described herein now permit functional interrogation of the ancestral molecular toolkit employed in the diversification of early animal body plans. Nematostella culture Nematostella adults were maintained in non-circulating 12 parts per thousand (p.p.t.) artificial seawater (sea salt; instant ocean) at 17 °C and were spawned every 3 weeks using a temperature of 28 °C and light intensity of 250–300 lumen per foot 2 for about 6 h [33] . Spawning occurs within 2–3 h after a cold-water change (17 °C). TALEN TALEN target sites were designed using TALEN Targeter [34] at https://tale-nt.cac.cornell.edu/ . TALEN plasmids were assembled according to the Golden Gate method [35] using the NN RVD modules. The final assembled TALEN repeats were ligated into the obligate heterodimer expression vectors [36] , pCS2TAL3-DD and pCS2TAL3-RR. TALEN mRNAs were synthesized using mMESSAGE mMACHINE SP6 kit (Life technologies) after linearization by NotI (New England BioLabs Inc.). The purification of mRNA was performed using a standard 3 M sodium acetate/ethanol precipitation protocol. mRNA quality was determined by a standard agarose gel electrophoresis. CRISPR/Cas9 gRNAs were designed with a previously described protocol [37] using the ZiFiT Targeter website ( http://zifit.partners.org/ ). The corresponding oligonucleotide pairs were annealed and cloned into the gRNA expression vector pDR274 (42250, Addgene) using BsaI. Primers are described in Supplementary Table 4 . gRNAs were in vitro transcribed using the MEGAshortscript T7 kit (Life Technologies) and DraI-digested pDR274 plasmid and purified using 3 M sodium acetate/ethanol precipitation. To test the CRISPR/Cas9 system in vitro , we used a recombinant Cas9 protein from Streptococcus pyogenes that contains 6 × His-tag and a nuclear localization signal (CP001, PNA Bio Inc.). This purified Cas9 protein (500 ng) was incubated with each gRNA (250 ng) and a linearized plasmid (450 ng) that contains 2 kb of NvFP-7R including exons 2 and 3. This reaction was performed in 1 × NEB buffer 3 with 1 × bovine serum albumin at 37 °C for 1 h. Following treatment with RNase, DNA fragments resulting from CRISPR/Cas9-induced cleavage were analysed by gel electrophoresis. For the expression of Cas9 from mRNA, we generated a PCR fragment encoding nlsEGFP-2A-Cas9 under the SP6 promoter. SP6-nlsEGFP-2A and Cas9-polyA were amplified from the pSYC-97 ref. 22 and pMLM3613 (42251, Addgene) plasmids, respectively, and assembled using the Gibson assembly Master Mix (E2611, New England BioLabs Inc.). The nlsEGFP-2A-mCherryCAAX construct was transcribed from pSYC-97 ref. 22 . Both nlsEGFP-2A-mCherryCAAX and nlsEGFP-2A-Cas9 mRNAs were synthesized using the mMESSAGE mMACHINE SP6 kit. Identification of Nematostella heat-shock-inducible promoters We identified five potential Nematostella HSP70 coding genes using a BLAST search against the Nematostella genome (Joint Genome Institute) and zebrafish HSP70 as a query. For each candidate heat-shock ( hs ) promoter, at least 1.5 kb DNA fragment upstream of the start codon was amplified from genomic DNA and cloned into a eGFP plasmid [38] using primers and restriction enzymes that are described in Supplementary Table 5 . The hs-eGFP constructs (20 ng μl −1 ) were individually injected into Nematostella eggs. To test their induction ability by heat shock, injected embryos were transferred to 1.5-ml eppendorf tubes in 500 μl artificial seawater and incubated at 37 °C for 30 min. Then, heat-shock-treated embryos were transferred to new culture dishes with fresh artificial seawater and were monitored every hour for eGFP expression under a dissecting scope. After 6–8 h post heat-shock treatment, the hs1 and hs2 promoters showed a strong and weak induction of eGFP expression, respectively. We used the hs1 promoter in all experiments. Construction of donor vectors Donor vectors were generated using the Gibson assembly Master Mix (E2611, New England BioLabs Inc). The backbone plasmids for the NvFP-7R::eGFP–MHC1-mCherry and hs-eGFP donor vectors were pHSG298 and pCS4+ plasmids, respectively. The hs-eGFP and homologous arms were, respectively, amplified from the plasmid described above and genomic DNA. The MHC1-mCherry construct is previously described [16] . Gibson assembly primers are listed in Supplementary Table 6 . Microinjection of Nematostella eggs Unfertilized eggs were dejellied in 4% cysteine (pH 7.4–7.6) for 10 min and washed three times in artificial seawater. Following dejellying, unfertilized eggs were injected using Femtojet Express (Eppendorf) during 2 h and then fertilized. For application of the CRISPR/Cas9 system with recombinant Cas9 protein, reaction mixtures (500 ng μl −1 Cas9 protein, 700 ng μl −1 gRNA-Exon2 and 70 ng μl −1 donor vector) were incubated at 37 °C for 10 min before injection to pre-assemble the gRNA–Cas9 complex. No incubation was necessary when 250 ng μl −1 nlsEGFP-2A-Cas9 mRNA was co-injected with 700 ng μl −1 gRNA-Exon2 and 70 ng μl −1 donor vector. TALEN- and CRISPR/Cas9-injected eggs were raised in the dark with daily water changes at 17 °C and room temperature, respectively. Genomic DNA extraction Genomic DNA was extracted from embryos or tissues that were surgically isolated from live polyps. Each sample was then incubated in 20 μl DNA extraction buffer (10 mM Tris-HCl pH 8, 50 mM KCl, 0.3% Tween 20, 0.3% NP40 and 1 mM EDTA) containing 1 μg μl −1 proteinase K at 58 °C for at least 5 h. Proteinase K was heat-inactivated by incubating the reaction at 98 °C for 20 min. We used 5 μl of genomic DNA extract for subsequent PCR analysis. Mutation analysis The genomic region containing the exon 2 of NvFP-7R was amplified from individual animal using specific primers: Exon2F 5′-GAATAACCAACAAATCTTTCTCTTTC-3′ and Exon2R 5′-TTGTCAACTTATCCTGTGAAATACCA-3′. Following sequencing, PCR products showing overlapping peaks in their chromatograms were cloned into pCR2.1/TOPO (Life Technologies) and then sequenced to confirm the presence of mutations at the target site. PCR analysis for genomic integration The primers used to amplify the sequence flanking the left (L) and right (R) homology arms of the eGFP–MHC-mCherry, hs - eGFP and MHC-mCherry cassettes were described in Supplementary Table 7 . PCR reactions were performed using Herculase II Fusion DNA polymerases (Agilent Technologies). Full-length images of agarose gels are shown in Supplementary Fig. 8 . Live imaging of Nematostella Following injection of nlsEGP-2A-Cas9 mRNA, embryos were mounted in a glass-bottom culture dish (MatTek corporation) using 1% low melting point agarose (SeaPlaque GTG Agarose, Lonza) and 12 p.p.t. artificial seawater. Time lapses were taken with a Zeiss LSM 700 using a Plan-Apochromat × 10 0.45 numerical aperture (NA) objective and 54-μm stacks (six slices) every 5 min with a 488-nm laser. Adult Nematostella were also imaged on a Zeiss LSM 780 with spectral imaging using a Fluar × 5 0.25 NA or a Plan-Apochromat × 10 0.45 NA. Control spectra were obtained separately for autofluorescence, eGFP and mCherry and then used for linear unmixing. Multi-day time lapses of adult polyps were obtained by imaging with a webcam controlled with Micro-Manager [39] . Animals were imaged during a 12 h dark/12 h light cycle after 2 days of acclimation. The InfraRed (IR) filter was removed to enable night imaging using IR light-emitting diodes. Light-induced contraction data were collected using Fiji [40] . How to cite this article : Ikmi, A. et al. TALEN and CRISPR/Cas9-mediated genome editing in the early-branching metazoan Nematostella vectensis . Nat. Commun. 5:5486 doi: 10.1038/ncomms6486 (2014).